An ultralow power athermal silicon modulator Silicon photonics has emerged as the leading candidate for implementing ultralow power wavelength–division–multiplexed communication networks in high-performance computers, yet current components (lasers, modulators, filters and detectors) consume too much power for the high-speed femtojoule-class links that ultimately will be required. Here we demonstrate and characterize the first modulator to achieve simultaneous high-speed (25 Gb s −1 ), low-voltage (0.5 V PP ) and efficient 0.9 fJ per bit error-free operation. This low-energy high-speed operation is enabled by a record electro-optic response, obtained in a vertical p – n junction device that at 250 pm V −1 (30 GHz V −1 ) is up to 10 times larger than prior demonstrations. In addition, this record electro-optic response is used to compensate for thermal drift over a 7.5 °C temperature range with little additional energy consumption (0.24 fJ per bit for a total energy consumption below 1.03 J per bit). The combined results of highly efficient modulation and electro-optic thermal compensation represent a new paradigm in modulator development and a major step towards single-digit femtojoule-class communications. Intra- and inter-chip interconnects, traditionally executed using parallel electrical links, are struggling to satisfy the current bandwidth, density, power consumption and cost requirements of the computing and communication industries [1] , [2] , [3] . These limitations are becoming apparent in rapidly scaling massively parallel computing systems such as data centers for cloud computing, and high-performance ‘supercomputers’ used for large-scale scientific computation. While current bottlenecks within the switches and interconnects of large-scale computing systems prove an immediate need for the inclusion of inter-chip optical components, on-chip (that is, intra-chip) communication links, where the bandwidth and efficiency requirements are far more severe, provide a long-term vision. An on-chip interconnecting wire that communicates one bit over an average distance of 1 mm (~10% of the die size), consumes 100 fJ per bit [4] . At the 8-nm node and beyond, over one petabit per second of data transfer will be required on large microprocessor die, leading to 100 W of communications power per chip (nearly 10 times what is acceptable in practice), and providing a clear motivation for on-chip photonic interconnects to be driven into the single-digit femtojoule per bit regime with each component within the link consuming just a fraction of that total [2] , [3] , [4] . Optical communications based on spatially division multiplexed vertical cavity surface emitting laser arrays already exist in high-performance computing systems [3] . Vertical cavity surface emitting laser-based links, which utilize multimode fibres, meet requirements in terms of cost and power consumption at low data rates (~100 Gb s −1 ). However, they are already struggling to satisfy future high-bandwidth (≥1Tb s −1 ), high-efficiency (~1 fJ per bit) requirements owing to their single-channel-per-fibre nature and multimode operation. A scalable alternative using wavelength division multiplexing is required. Wavelength division multiplexing systems offer high-bandwidth operation per fibre, and can be efficiently implemented by using on-chip silicon photonic modulators to encode data on a laser comb. Silicon photonics [5] , inherently complementary metal-oxide semiconductor (CMOS) compatible, offers a high-index contrast platform that allows for single-mode high-confinement waveguides that lead to compact resonators and high-speed, low-energy consumption modulation [6] . In the silicon platform, high-performance electro-absorptive germanium-on-silicon and electro-refractive silicon modulators have been demonstrated [7] , [8] , [9] , [10] , [11] , [12] , [13] , [14] , [15] , [16] , [17] , [18] , [19] , [20] . Germanium-on-silicon modulators use the strong Franz–Keldysh and Quantum-confined Stark effects, and have enabled low-power non-resonant modulators [7] , [8] . However, electro-absorption devices also act as detectors and the generated photocurrent leads to an additional, significant term in the power consumption of the modulator [21] . Further, in order to achieve a large extinction ratio (ER), all germanium-on-silicon electro-absorption modulators to date have required voltage levels that are not compatible with CMOS drive levels. Finally, since electro-absorption devices are based on a band-edge effect, the material composition inherently limits the operation to a modest wavelength range. The band-edge can be engineered to enable wideband operation, but only at the expense of additional mask layers, regrowth and fabrication complexity. In contrast, silicon modulators employ the relatively weak free-carrier plasma dispersion effect [22] , which induces a change in carrier concentration to alter the refractive index in the device. The index change results in a phase shift, which can be translated into an amplitude response using a Mach–Zehnder interferometer or a resonant cavity. Early on-chip demonstrations of silicon modulators used poorly confined ridge waveguides to form large Mach–Zehnder interferometers (>500 μm in length) and were inefficient due to large drive voltages and/or currents and high device capacitance [9] , [10] . In order to enhance the electro-optic effect, high-confinement, compact silicon resonant structures were proposed. Resonant modulators confine light in high-quality factor ( Q ) devices that effectively increase the optical path length and, thus, the interaction with the modulated carrier distribution. Compact devices also minimize the total device capacitance, enabling high-speed and low-power operation. Xu et al. [11] demonstrated the first silicon resonant electro-optic modulator using injection of carriers in a p – i – n junction diode. A variety of silicon resonant modulators have since been demonstrated [13] , [14] , [15] , [16] , [17] , [18] , [19] , [20] . Injection-based modulators have achieved large frequency shifts, but at the expense of low-speed operation (~1.5 Gb s −1 ) due to the long free-carrier lifetime (τ~1 ns) within silicon diodes. Signal pre-emphasis has been used to achieve high-speed operation, but at the expense of increased power consumption and CMOS complexity [12] . In order to overcome these limitations, resonant silicon modulators based on the depletion of electrons and holes have been realized and have achieved innate low-energy, low-voltage and high-bandwidth operation [13] , [14] , [15] , [16] , [17] , [18] , [19] , [20] . The first depletion-based resonant modulator utilized a vertical p – n junction and achieved an error-free energy per bit of just 60 fJ per bit, paving the way for ultralow power modulators [13] . The vertical junction enabled interior p+ and n+ contacts, eliminating the need for a ridge waveguide, and preserving the hard outer wall of a step-index silicon microdisk. The hard outer wall yielded better modal confinement, allowing for more compact (~3.5 μm diameter) microdisk modulators, with larger free spectral ranges and greatly reduced total device capacitance [13] , [14] , [15] , [16] . In addition, the vertical junction microdisk modulators exhibit a much larger overlap of the junction with the optical mode, a result characterized by the junction capacitance per unit volume (as discussed in the Results section), enabling electro-optic responses as large as 60 pm V −1 (7.5 GHz V −1 ) (ref. 14 ) and 90 pm V −1 (11 GHz V −1 ) [15] . Driven in both depletion and sub-threshold forward-biased modes, these microdisk modulators achieved an error-free energy per bit of just 3 fJ at 12.5 Gb s −1 (ref. 14 ) and, an error-free ~13 fJ per bit modulation up to 25 Gb s −1 (ref. 15 ). These modulators have a device capacitance of 12 fF in a 1.6-μm 3 junction volume [14] and a device capacitance of 36 fF in a 4.6-μm 3 junction volume [15] . The electro-optic responses were correlated with the junction capacitance per unit volume, which will be verified in the following paragraphs. When driven differentially, these modulators achieved an error-free energy per bit of just 0.9 fJ per bit at a data rate of 10 Gb s −1 (ref. 16 ). Despite the low-power operation of vertical junction modulators, ridge-based microring modulators with lateral junctions and interior and exterior contacts have persisted owing to their ease of implementation. Early demonstrations of ridge-based depletion modulators achieved operation at 10 Gb s −1 with an energy per bit of ~50 fJ per bit, an electro-optic response of 20 pm V −1 (~2.5 GHz V −1 ) and a device capacitance of 50 fF in an 11.6-μm 3 junction volume [17] . More recent ridge-waveguide-based microring modulators using lateral junctions have achieved an energy consumption of ~7 fJ per bit, an electro-optic response of 26 pm V −1 (~3 GHz V −1 ) and a junction capacitance of 20.5 fF in a 5.4-μm 3 junction volume [18] . However, no bit error rate information was provided. Other demonstrations at 25 Gb s −1 have also been made using interleaved junctions with 471 fJ per bit, an electro-optic response of 34 pm V −1 (~4 GHz V −1 ), and a device capacitance of 184 fF in a 33.1-μm 3 junction volume [19] and >66 fJ per bit without bit error rate (BER) information and with an electro-optic response of 40 pm V −1 (~5 GHz V −1 ) and a junction capacitance of 66 fF in a 28.3-μm 3 junction volume [20] , thus highlighting the challenge of achieving low-energy error-free operation at high data rates. Yet, future communication links are expected to run at 25 Gb s −1 . The difficulty in realizing high data rates in resonant modulators lies in the fact that, in bandwidth-limited modulators, operation at 25 Gb s −1 requires an electro-optic shift that is 2.5 times larger than at 10 Gb s −1 in order to sustain the performance (for example, insertion loss (IL) and extinction ratio (ER)). Given the square root dependence of the depletion width with applied voltage, doing so requires 6.25 times the voltage, resulting in ~39 times more energy per bit ( E bit = CV 2 /4) than is required at 10 Gb s −1 . While some of the aforementioned results are impressive, none have achieved single-digit femtojoule-class communications at the high data rates that will be required in future on-chip communication links and all results thus far have been achieved in thermally stable environments that are not representative of a real application. In this work, we present the design and demonstration of an athermal resonant silicon modulator that is compatible with a CMOS process, operates at high data rates and achieves the lowest total energy per bit performance to date. These results are made possible by combining interior circular contacts and a highly optimized vertical junction within a compact microdisk modulator. The circular contacting scheme enables a direct, short electrical path out to the vertical junction, minimizing the resistance and corresponding loss in depletion/accumulation response and maximizing the speed of the modulator. The vertical junction profile optimizes the optical mode overlap and maximizes capacitance per unit volume. As a result, we achieve a record 250 pm V −1 (30 GHz V −1 ) electro-optic frequency response and, thus simultaneous error-free, high-speed (25 Gb s −1 ), low-voltage (0.5 V PP ) and low energy per bit (0.9 fJ per bit) operation. Not only does the large electro-optic response allow for sub-1 fJ per bit operation, but it also simultaneously improves the IL and ER compared with prior demonstrations [13] , [14] , [15] , [16] , [17] , [18] , [19] , [20] . Further, the record electro-optic frequency response can be used to counteract thermal shifts over a 7.5 °C (~75 GHz) temperature (frequency) range by varying the DC bias point of the modulator. This adds little additional energy consumption (only 0.24 fJ per bit due to leakage current), while modulation energy decreased to 0.79 fJ per bit, enabling 1.03 fJ per bit athermal operation. Over a 10 °C temperature range, the modulator consumes 0.77 fJ per bit modulation energy and an additional 2 fJ per bit due to undesired leakage current, resulting in 2.77 fJ per bit total energy consumption. Finally, while these demonstrations were all performed at 25 Gb s −1 , the modulator demonstrates open-eye diagrams at data rates as high as 44 Gb s −1 when driven with higher voltages. Optimizing a depletion-mode modulator In a resonant depletion-mode modulator, a voltage applied to a p – n junction changes the depletion width, which, through the plasma dispersion effect, results in a perturbation to the permittivity (Δε) [22] . This permittivity change induces a resonant frequency shift to each mode m of Δ ω m . The magnitude of the shift can be derived from Poynting’s theorem and is expressed as the ratio between the perturbed and total energy within the resonator [23] . where, ε is the permittivity of silicon, ω m the unperturbed resonant frequency, e m the electric field distribution of mode number m , and ν p and ν o are the perturbed and total resonator volume, respectively. The approximation assumes the electric field, e m , has a uniform flattop distribution within the silicon core. Furthermore, the total resonator volume can be approximated by ν o = WHL , where W , H and L are the width, height and length of the resonator core, respectively. Similarly, the perturbed volume is approximated by ν p =Δ w d DL , where Δ w d is the change in depletion region size at a given applied potential, D is a junction-profile-dependent parameter, which is shown in Fig. 1a and L is the length of the resonator. D is equal to H in lateral [17] , [18] and W in vertical [13] , [14] , [15] , [16] junction profiles, and to the ratio of the core area ( HW ) to half the length of the p – n junction period, L p–n , ( D =2 HW / L p–n ) for an interleaved junction profile [19] , [20] . The relative change in permittivity (Δ ε / ε ) is related to the relative change in refractive index (Δ n/n ) by Δ ε / ε =(( n+ Δ n ) 2 − n 2 )/ n 2 ≈2Δ n / n . 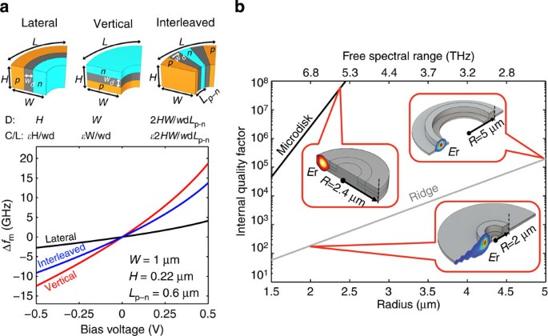Figure 1: Junction profile comparison. (a) The lateral, vertical and interleaved junction profiles are illustrated for common depletion-mode modulators. The capacitance per unit length (C/L) is expressed below each junction profile. Frequency shifts based on equations (2), (3) and (6) are calculated as a function of applied potential for lateral, vertical and interleaved junction profiles, showing the large frequency shift of vertical junction profile. Calculations were performed atλ=1.55 μm and for a built-in potential of 0.7 V and a n- and p-type carrier concentration of 3 × 1018cm−3. (b) The internal quality factors are plotted as a function of radius for an undoped microdisk and ridge resonators, showing high confinement and quality factor for the microdisk resonator. The TE radial mode profiles are overlaid with the resonator cross-sections. The thickness of the microdisk resonator was 220 nm. The ridge resonator had the crossection of the modulator in ref.18. Substituting into equation (1) gives: Figure 1: Junction profile comparison. ( a ) The lateral, vertical and interleaved junction profiles are illustrated for common depletion-mode modulators. The capacitance per unit length (C/L) is expressed below each junction profile. Frequency shifts based on equations (2), (3) and (6) are calculated as a function of applied potential for lateral, vertical and interleaved junction profiles, showing the large frequency shift of vertical junction profile. Calculations were performed at λ =1.55 μm and for a built-in potential of 0.7 V and a n- and p-type carrier concentration of 3 × 10 18 cm −3 . ( b ) The internal quality factors are plotted as a function of radius for an undoped microdisk and ridge resonators, showing high confinement and quality factor for the microdisk resonator. The TE radial mode profiles are overlaid with the resonator cross-sections. The thickness of the microdisk resonator was 220 nm. The ridge resonator had the crossection of the modulator in ref. 18 . Full size image Equation (2) can be further simplified by relating the change in refractive index (Δ n ) to the acceptor- and donor-free carrier concentrations through a curve fit [22] to Soref’s experimental data in [14] . where, N D and N A are the donor and acceptor concentrations, respectively, and the curve fitting parameters for donors and acceptors are A D =−2.37 × 10 −23 , B D =1.08, C D =4.92 × 10 −26 , D D =1.2, and A A =−3.93 × 10 −18 , B A =0.772, C A =1.96 × 10 −24 , D A =1.1. Note that the imaginary part of the index change modifies the cavity loss but does not induce a real frequency shift. It is therefore the real part of the index change that matters in equation (2). Assuming, for simplicity, that B A ≈ B D ≈1, A≈A A ≈A D and N A ≈ N D ≈ N, equation (2) can be rewritten as: Finally, the depletion width change can be related to the device capacitance through the accumulated charge by considering Δ Q/L = qND Δ w d (where q is the electronic charge) and Δ Q≈C Δ V=CV pp for Δ w d << w d , where V is the applied electric potential and C is the junction capacitance, εDL/w d . The final result is then: We, thus conclude that, to first order, the frequency shift of a depletion-based modulator is directly proportional to the capacitance per unit volume of the resonator ( C/v o ). Since the waveguide cross-section is generally fixed to maintain single-mode operation, it is desirable to maximize the junction capacitance per unit length to achieve the largest frequency shift. It is important to note that the depletion width and junction capacitance are a function of the applied potential. The approximate depletion width for an abrupt p – n junction as a function of voltage is given in equation (6): assuming N A ≈ N D ≈ N and where φ B is the built-in potential [24] . The vertical junction in our modulator serves to maximize the capacitance per unit volume and thereby ensures maximal frequency shift for a given applied voltage. To illustrate the advantage of a vertical junction over the typical interleaved or lateral junctions, the resonant frequency shifts as a function of voltage are calculated using equations (2), (3) and (6), and depicted in Fig. 1a . As can be seen, the vertical junction profile provides a much larger frequency shift (Δ f vertical ~30.9 GHz V −1 ) at a given applied voltage than the lateral (Δ f lateral ~6.9 GHz V −1 ) or the interleaved (Δ f interleaved ~22.7 GHz V −1 ) profiles. To achieve a given frequency shift, the vertical junction profile thus requires 4.5 and 1.4 times smaller voltage drive, respectively, which translates to ~20 and ~2 times smaller energy consumption (switching energy, E s = CV 2 ) [21] . Note also that the electro-optic response of the current vertical junction profile is larger than that in [13] , [14] , [15] , [16] , [25] owing to improvements in device geometry and doping concentration, as indicated above. However, while increasing the capacitance per unit volume in the optically active region of the resonator is helpful, reducing the overall capacitance of the device is desired to achieve the lowest switching energy. The use of an interior circular contact together with a hard outer resonator wall in the microdisk aids in doing just that by allowing for a tightly confined, compact device as shown in Figs 1b and 2a . Compared with a typical ridge-waveguide-based resonator, the overall resonator volume is minimized and the capacitance is concentrated over the optically active region of the junction as shown in Fig. 1b . The quality factor of an undoped microdisk resonator with a radius of 1.5 μm is equivalent to that of an undoped ridge resonator with a radius of 4.5 μm. The sharp bending radius of microdisk resonator leads to >9 times less volume when it is compared with the typical ridge-contacted microring resonator. In addition, the interior circular contact, enabled by overlapping p+ and n+ regions within the microdisk center, also minimizes the device resistance. This is the first time such a contact has been realized within any silicon modulator. Minimizing the resistance allows for the applied voltage to be dropped directly across the optically active region of the junction, significantly improving performance as only radial- and vertical-resistive components, illustrated in Fig. 2a , are relevant, and the large azimuthal resistances, which limited the performance of prior demonstrations [13] , [14] , [16] , [25] , are eliminated. Given the very short electrical paths to the vertical junction there is effectively no parasitic resistance to inhibit the electro-optic response or the bandwidth , enabling much higher performance than previously possible. The low resistance and smaller overall capacitance, together with the large capacitance per unit volume, make this modulator a significant advance over prior geometries [11] , [12] , [13] , [14] , [15] , [16] , [17] , [18] , [19] , [20] . 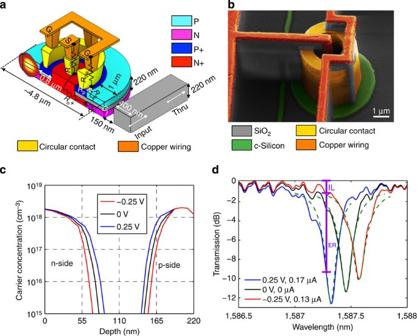Figure 2: Silicon vertical junction microdisk modulator design and characterization. (a) A three-dimensional sketch of the electro-optic silicon microdisk modulator, showing the cross-section, size, metal connections and the optical mode overlapped with the vertical p–n junction. The grey regions illustrate the depletion region in the vertical p–n junction within the microdisk and the undoped bus waveguide adjacent to the microdisk. The full doping profile, including the n+ and p+ regions as well as all of the wiring shown in the diagram was included in all calculations. The electrical equivalent diagram of the circularly contacted microdisk is also overlaid, illustrating n+, p+, p, n-doped region and vertical via resistances (Rn+,Rp+,Rp,Rn andRvia) as well as the junction capacitance (Cj). Owing to its cylindrical symmetry, the device has only vertical and radial resistance terms and no azimuthal resistance term, which significantly reduces the contact and device resistance. (b) A scanning electron microscopy image of the silicon microdisk modulator, revealed by dry etching the SiO2around the modulator to show the metal interconnect, circular contact, silicon bus waveguide and the microdisk. The signal pad, connected by short (~10–100μm) wires, is shown on the left side of the image. (c) The simulated finite element model (FEM) vertical junction carrier distribution profile is plotted as a function of applied voltage and depth. (d) The measured and simulated (green dashed curves) transmission spectra of the resonator is plotted, at ~26.5 °C and with applied DC bias voltages of 0.25, 0 and −0.25 V, respectively. Figure 2: Silicon vertical junction microdisk modulator design and characterization. ( a ) A three-dimensional sketch of the electro-optic silicon microdisk modulator, showing the cross-section, size, metal connections and the optical mode overlapped with the vertical p – n junction. The grey regions illustrate the depletion region in the vertical p–n junction within the microdisk and the undoped bus waveguide adjacent to the microdisk. The full doping profile, including the n+ and p+ regions as well as all of the wiring shown in the diagram was included in all calculations. The electrical equivalent diagram of the circularly contacted microdisk is also overlaid, illustrating n+, p+, p, n-doped region and vertical via resistances ( R n+ , R p+ , R p , R n and R via ) as well as the junction capacitance ( C j ). Owing to its cylindrical symmetry, the device has only vertical and radial resistance terms and no azimuthal resistance term, which significantly reduces the contact and device resistance. ( b ) A scanning electron microscopy image of the silicon microdisk modulator, revealed by dry etching the SiO 2 around the modulator to show the metal interconnect, circular contact, silicon bus waveguide and the microdisk. The signal pad, connected by short (~10–100μm) wires, is shown on the left side of the image. ( c ) The simulated finite element model (FEM) vertical junction carrier distribution profile is plotted as a function of applied voltage and depth. ( d ) The measured and simulated (green dashed curves) transmission spectra of the resonator is plotted, at ~26.5 °C and with applied DC bias voltages of 0.25, 0 and −0.25 V, respectively. Full size image Designing a vertical junction microdisk modulator The microdisk modulator, including the fabrication process steps (see the Methods section for details), was simulated using Synopsys’s Sentaurus software suite, and the carrier concentration as a function of voltage was extracted and is shown in Fig. 2c . In this graph, the energies of the implants that form the vertical junction have been slightly adjusted to fit the experimental voltage vs spectral response curves (see the fabrication part of the Methods section for details). The depletion width can be approximated as the distance between 50% of the peak of the n and p doping concentrations. Using this approximation, the depletion width is estimated to be 124, 132 and 139 nm for applied voltages of 0.25, 0 and −0.25 V, respectively. The radial electric field component of the optical mode, simulated using a complex, full-vectorial and cylindrical finite difference mode solver (FDM) [26] , is shown in Fig. 2a . As can be seen, there is a large modal overlap between the vertical depletion region and the optical mode yielding a large frequency shift. In order to ensure high- Q operation, the highly doped p+ and n+ regions, which act as low-resistance contacts, were placed 1 μm away from the outer wall of the resonator where there is only negligible overlap with the optical mode. The cylindrical FDM simulations show that the 220-nm-thick silicon microdisk with its hard outer resonator wall supports a radiation-limited internal Q of over one million for diameters as small as 4 μm. Here, we chose a 4.8-μm diameter microdisk owing to contact geometry and process design rule limitations, as opposed to radiation limits, which resulted in a 2.5-μm 3 junction volume. The capacitance of the modulator ( C = Q / V ), including the full doping profile, n+ and p+ regions and the wiring shown in Fig. 2a–c , was estimated to be ~17 fF from AC Sentaurus device simulations. The compact junction volume combined with the vertical junction and the circular contact maximize capacitance per unit volume and minimize total device capacitance and device resistance. This modulator consumes an estimated switching energy ( E s = CV 2 ) of ~4.25 fJ for an AC-coupled 0.5 V PP drive voltage. In a non-return-to-zero (NRZ) pseudo-random bit sequence (PRBS) signal, the 0–0, 0–1, 1–0 and 1–1 transitions are equally probable (p(0–0)=p(0–1)=p(1–1)=p(1–0)=1/4), and the modulator only consumes energy from the source in the 0-1 transitions ( E 0–1 = E s, E 0–0 =0, E 1–1 =0, E 1–0 =0). Therefore, the estimated energy per bit ( E bit =p(0–0) × E 0–0 +p(0–1) × E 0–1 +p(1–1) × E 1–1 +p(1–0) × E 1–0 = E s /4= CV 2 /4) is 1.06 fJ per bit. An electrical step function from −0.25 to 0.25 V was applied in the Sentaurus device simulation to the modulator, including the full doping profile and the wiring shown in Fig. 2a . The resultant step response was fitted with an exponential rise function, revealing an estimated electrical 3 dB bandwidth of ~35 GHz. Characterizing the DC optical response A continuous-wave lightwave generated by a tunable laser source was coupled to the fundamental transverse-electric (TE)-mode of the on-chip silicon waveguide using a tapered single-mode fibre. The through port spectral response as a function of applied DC bias was measured at a temperatue of 26.5 °C and the results are plotted in Fig. 2d alongside the numerical simulations (see the Methods section for details). The loss within the modulator was both measured and simulated to be ~29 dB cm −1 . Losses from radiation and sidewall roughness are found to be negligible compared with the loss from free-carrier absorption. The p–n junction acts as a capacitor in the reverse-biased and sub-threshold forward-biased regimes of operation. Frequency shifts of +8 and −7 GHz, resulting from the charging and discharging of this capacitor, were observed under applied biases of 0.25 and −0.25 V, respectively. These shifts agree well with the theoretical predictions and reveal a record 250 pm V −1 (30 GHz V −1 ) response. The optical modulation bandwidth can be extracted from the full-width-half-maximum and is equal to: [27] . The factor stems from the fact that the resonator stores light (to achieve data level 0) and releases the light (to achieve data level 1). The full-width-half-maximum was measured to be ~30 GHz (see Fig. 2d ), which yields an optical modulation bandwidth of ~19.3 GHz. Combined with the simulated electrical modulation bandwidth (~35 GHz, see above), this yields a device bandwidth, , of ~17 GHz, calculated using . Measuring modulation energy consumption The electrical power and switching energy of the stand-alone modulator were measured using a time domain reflectometer (TDR) (see the Methods section for details). The measurement, shown in Fig. 3c , is performed for an AC-coupled 0.5 V PP drive dropped across the modulator via a 50 Ω terminated probe. The probe is terminated because without the termination, only a ~0.25 V PP drive is required due to the large reflection that would otherwise occur at the high-impedance modulator. However, the modulator is intended to operate with an integrated CMOS circuit, which will drop the drive voltage across the modulator pins without reflection since the circuit is connected by a local deep sub-wavelength electrical interconnnect and transmission line effects are not present. Thus, the 50-Ω termination is required to accurately characterize the modulator performance under the intended method of operation, but it will be neither used nor required in practice. The switching energy and energy per bit of the microdisk were experimentally extracted (see the Methods section for details) to be 3.65 and 0.91 fJ per bit, respectively, which agrees well with the simulated values. The slight difference between the theoretical and experimental results can be explained by a slightly lower p+ and n+ implant activation compared with the simulations, which would reduce the overall device capacitance. Wire and/or pad capacitance add to the device capacitance. However, with both direct integration and advanced three-dimensional integration techniques this addition can be quite low. For example, in direct integration the total via/wire capacitance has been estimated to be 5 fF (ref. 28 ). In wafer bonding based on three-dimensional integrated through-oxide-vias [29] , the via capacitance has been measured to be ~2 fF. Therefore with through-oxide-vias, the ground and signal vias will add a total of 4 fF of capacitance, similar to the direct integration case. In either case, the parasitic capacitance will add only ~0.3 fJ per bit, and the modulator energy consumption will still stay close to 1 fJ per bit. 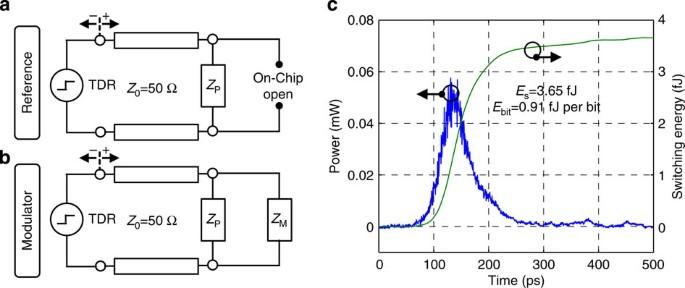Figure 3: Energy consumption. (a) The electrical setup for the time domain reflectometry (TDR) reference measurement, configured for measuring the reflected voltage (VP−) from the open-ended on-chip pads (ZP). (b) The electrical setup for the TDR reference and modulator measurement, configured for measuring the reflected voltage (VPM−), from the modulator load (ZM) and identical on-chip pads (ZP). The TDR input and reflected TDR output directions are depicted with+and − signs. (c) The TDR measurement of the electro-optic modulator power consumption and switching energy for a 0.5-VPPAC-coupled drive. Figure 3: Energy consumption. ( a ) The electrical setup for the time domain reflectometry (TDR) reference measurement, configured for measuring the reflected voltage ( V P − ) from the open-ended on-chip pads ( Z P ). ( b ) The electrical setup for the TDR reference and modulator measurement, configured for measuring the reflected voltage ( V PM − ), from the modulator load ( Z M ) and identical on-chip pads ( Z P ). The TDR input and reflected TDR output directions are depicted with+and − signs. ( c ) The TDR measurement of the electro-optic modulator power consumption and switching energy for a 0.5- V PP AC-coupled drive. Full size image Demonstrating high-speed and error-free transmission High-speed optical eye diagrams, shown in Fig. 4a , were measured using a high-speed electro-optic setup (see the Methods section for details) with a digital sampling oscilloscope at data rates of 10, 15, 20 and 25 Gb s −1 . The dynamic ER and IL are shown below each eye diagram in Fig. 4a . The dynamic ER is defined as the ratio of the average data level 1, ‹1›, and the average data level 0, ‹0›, ER=10log(‹1›/‹0›). The IL, illustrated in Fig. 4a , is defined as the difference between the average data level 1, ‹1›, and the optical true ‘1’ as given by the off-resonance intensity at λ ~1,588 nm: IL=10log((‹1›−‹0›)/(1−‹0›)). Note also that the optical true ‘0’ corresponds to the amplified spontaneous emission floor after the filter at λ ~1,588 nm. The modulator exhibits low IL (~1.0 dB) and a high ER (6.2 dB) at a data rate of 25 Gb s −1 for 0.5 V PP drive voltage. The increased IL at high data rates can be explained by the electro-optic bandwidth limitation. 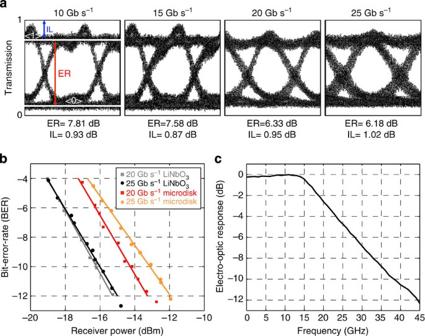Figure 4: High-speed modulator characterization. (a) The experimentally measured high-speed optical eye diagrams of the silicon electro-optic modulator driven by a terminated probe and 0.5 VPPNRZ-OOK PRBS with a pattern length of 231-1 at data rates of 10-, 15-, 20- and 25-Gb s−1. The extinction ratio (ER) and insertion loss (IL) are denoted below the eye diagrams at each data rate. (b) The bit error rate curves measured for the silicon microdisk and commercial LiNbO3modulators, for 20- and 25-Gb s−1data rates. The bit error rate curves for the commercial LiNbO3modulator were used as a reference to obtain the power penalty of the silicon microdisk modulator. (c) The electro-optic frequency response of the silicon modulator. Figure 4: High-speed modulator characterization. ( a ) The experimentally measured high-speed optical eye diagrams of the silicon electro-optic modulator driven by a terminated probe and 0.5 V PP NRZ-OOK PRBS with a pattern length of 2 31 -1 at data rates of 10-, 15-, 20- and 25-Gb s −1 . The extinction ratio (ER) and insertion loss (IL) are denoted below the eye diagrams at each data rate. ( b ) The bit error rate curves measured for the silicon microdisk and commercial LiNbO 3 modulators, for 20- and 25-Gb s −1 data rates. The bit error rate curves for the commercial LiNbO 3 modulator were used as a reference to obtain the power penalty of the silicon microdisk modulator. ( c ) The electro-optic frequency response of the silicon modulator. Full size image In order to further quantify the modulator performance, bit-error-rate (BER) measurements, shown in Fig. 4b , were performed at data rates of 20 and 25 Gb s −1 . For data rates up to 25 Gb s −1 , the device achieves error-free operation (BER <10 −12 ) for a PRBS pattern length of 2 31 −1. We did not observe any pattern length dependence on the BER with pattern lengths ranging from 2 7 −1 to 2 31 −1. This is owing to the use of depletion-mode operation and extremely low drive voltages, and the low power consumption of the device limiting the thermal load on the device, which normally contributes to long-pattern errors [30] . A commercial LiNbO 3 Mach–Zehnder modulator was similarly characterized for reference. The commercial modulator is rated to a 3 dB bandwidth of 35 GHz, and driven with an AC-coupled 5.5 V PP electrical signal. The power penalty was recorded as the received power difference at a BER of 10 −12 between the silicon microdisk modulator and the commercial LiNbO 3 modulator, as depicted in Fig. 4b . Data transmission with the silicon microdisk modulator was received with a power penalty of 3.0 and 3.06 dB at data rates of 20 and 25 Gb s −1 , respectively. The increased power penalty at high data rates can be explained by the electro-optic bandwidth difference between the two modulators and the phase chirp that is introduced by the resonant modulator. Measuring electro-optic bandwidth The electro-optic response of the modulator was characterized using an electrical signal source with a frequency range from DC to 50 GHz. The electrical signal output was calibrated to achieve a constant peak-to-peak drive voltage for the entire frequency span. The laser was then aligned to the highly linear part of the resonance at λ ~1,578.4 nm and a 50 mV PP sinusoidal small-signal was applied to the microdisk modulator at frequencies spanning 500 MHz to 45 GHz. The through port power was measured with an external p–i – n photodiode and transimpedance amplifier receiver. The peak-to-peak AC level was recorded and plotted in Fig. 4c . The electro-optic 3 dB bandwidth was experimentally measured to be ~21 GHz, which agrees well with our theoretical small-signal estimate of 17 GHz. The difference is largely owing to the fact that the theoretical estimate was calculated for on-resonance operation and the modulator electro-optic bandwidth was measured slightly off-resonance to preserve linearity and to achieve a faster response, similar to [31] . Exhibiting thermal compensation by electro-optic tuning The baseline electro-optic response of this modulator, 250 pm V −1 (30 GHz V −1 ), enables 1 fJ per bit operation at 25 Gb s −1 , represents a new standard for resonant modulators. More importantly, the electro-optic response is sufficiently large to compensate for thermal shifts up to 10 °C. Here, we demonstrate this principle by varying the temperature of the chip from 20–30 °C (see the Methods section for details) and compensating for that variation with electro-optic tuning achieved by varying the bias voltage from −2.2 to 0.4 V. The through port spectral response as a function of applied DC bias was measured at ~26.5 °C and the results are plotted in Fig. 5a . The modulator shifts ~100 GHz over an applied voltage range from −2.2 to 0.4 V. The resonant modulator spectra without and with electro-optic thermal compensation over a temperature range of 20–30 °C are shown in Fig. 5b,c , respectively. The resonance is tuned electro-optically by utilizing the free-carrier plasma dispersion effect rather than through traditional thermo-optic tuning. The p–n junction acts as a capacitor in the reverse-biased and sub-threshold forward-biased regimes of operation. The electro-optic tuning consumes energy only if the transitions charge the capacitor. Given a microprocessor thermal time constant of τ ≫ 1 μs [32] , a worst-case electro-optic tuning power of 69.6 nW ( P s = CV 2 /τ=69.6 fJ 1 −1 μs=69.6 nW) where C is determined from TDR measurements (see the Methods section for details), is required, resulting in a negligible energy per bit of 0.28 aJ per bit ( E bit =69.6 nW/25 Gb s −1 =0.28 aJ per bit), shown in Fig. 5g . Up to 27.5 °C, the leakage current was sufficiently low that it contributed an additional tuning energy of only 0.24 fJ per bit. Therefore, the modulator operated over a 7.5 °C range with 1.03 fJ per bit energy consumption including both tuning (0.24 fJ per bit) and modulation energy (0.79 fJ per bit). The modulation energy is slightly decreased owing to the widened depletion region at the reverse-biased operation (equation (6)) that reduced the device capacitance, as shown in Fig. 5f,g . To achieve a full 10 °C temperature range, a −2.2 V bias is required, resulting in a leakage current of 23 μA, and consuming a static power of 50.6 μW. This corresponds to an additional energy cost of 2 fJ per bit, while modulation energy was reduced to 0.77 fJ per bit. The compensating frequency shift originates primarily from electro-optic tuning with a minor contribution from thermo-optic tuning due to the high leakage current resulting from undesired band-to-band tunnelling between the highly doped contact regions at the larger reverse biases, which can be mitigated with process optimization. The undesired leakage current also contributed to a small thermo-optic resonance frequency shift of ~7.2 GHz (Δ f ≈ IV /7 μW GHz −1 =7.2 GHz [25] ). While tuning the resonance appropriately for the given temperature, the modulator was driven by a terminated 0.5 V PP drive with a PRBS length of 2 31 -1 at a data rate of 25 Gb s −1 across the 10 °C temperature range while observing negligible degradation in eye diagrams and/or error rate. The resulting high-speed optical eye diagrams, shown in Fig. 5e , were measured using a digital sampling scope. The high ER and low IL were preserved over the 10 °C temperature range at 25 Gb s −1 transmission. BER measurements, shown in Fig. 5d , were performed at a data rate of 25 Gb s −1 and the modulator achieves error-free operation (BER <10 −12 ) for a PRBS pattern length of 2 31 −1 over the 10 °C temperature range. The power penalty of the data transmission at a BER of 10 −12 due to thermal variations was within ±0.14 dB. The total energy consumption, shown on Fig. 5f-g for each case, was determined to be 1.03 fJ per bit over a 7.5 °C temperature range and 2.77 fJ per bit over a 10 °C temperature range. All prior demonstrations of resonant silicon modulators required thermo-optic tuning owing to their relatively small electro-optic frequency responses. However, implementing thermal tuning within modulators requires additional contacts, complicating and often degrading the modulator performance. When tuned over a 10 °C temperature range, the energy consumption of these devices increased substantially to ~82 fJ per bit (7 μW GHz −1 × 100 GHz/10 10 bits s −1 +12 fJ per bit=82 fJ per bit) [25] and ~175 fJ per bit (42 μW GHz −1 × 100 GHz/(2.5 × 10 10 bits s −1 )+7 fJ per bit=175 fJ per bit) [18] at data rates of 10 and 25 Gb s −1 , respectively. 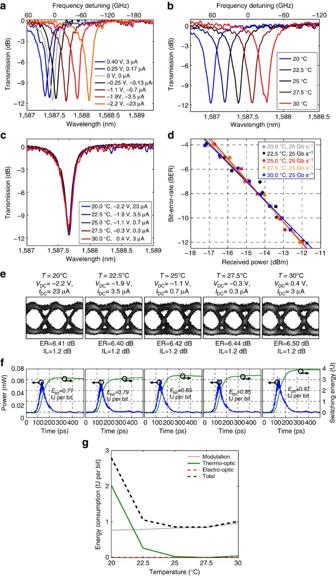Figure 5: Temperature-insensivitive operation. (a) The measured transmission spectra of the resonant modulator at ~26.5 °C and applied DC bias voltages ranging from 0.4 to −2.2 V. (b) The measured transmission spectra of the resonant modulator over a 10 °C temperature range at 0 V applied bias. The thermo-optic frequency response was extracted to be ~10 GHz per °C. (c) The measured transmission spectra of the resonator over a 10 °C temperature range with the modulator tuned electro-optically to compensate for thermal variations. (d) The bit error rate curves measured over a 10 °C temperature range for the silicon resonant modulator, driven by a terminated probe and 0.5 VPPNRZ-OOK PRBS with a pattern length of 231-1 at a data rate of 25 Gb s−1. The bit error rate curves clearly show error-free operation over the 10 °C temperature range. (e) Experimentally measured high-speed optical eye diagrams of the silicon electro-optic modulator at a data rate of 25 Gb s−1. The applied bias voltage (VDC) and measured current (IDC) are denoted above the eye diagrams at each temperature. The extinction ratio (ER) and insertion loss (IL) are denoted below the eye diagrams at each data rate and temperature. (f) The TDR measurement of the electro-optic modulator energy consumption and switching energy for a 0.5 VPPdrive is shown for the indicated DC bias voltages. (g) The breakdown of the thermo-optic, electro-optic and total modulator energy consumption is plotted as a function of temperature, showing the 1 fJ bit operation over 7.5 °C temperature range. Figure 5: Temperature-insensivitive operation. ( a ) The measured transmission spectra of the resonant modulator at ~26.5 °C and applied DC bias voltages ranging from 0.4 to −2.2 V. ( b ) The measured transmission spectra of the resonant modulator over a 10 °C temperature range at 0 V applied bias. The thermo-optic frequency response was extracted to be ~10 GHz per °C. ( c ) The measured transmission spectra of the resonator over a 10 °C temperature range with the modulator tuned electro-optically to compensate for thermal variations. ( d ) The bit error rate curves measured over a 10 °C temperature range for the silicon resonant modulator, driven by a terminated probe and 0.5 V PP NRZ-OOK PRBS with a pattern length of 2 31 -1 at a data rate of 25 Gb s −1 . The bit error rate curves clearly show error-free operation over the 10 °C temperature range. ( e ) Experimentally measured high-speed optical eye diagrams of the silicon electro-optic modulator at a data rate of 25 Gb s −1 . The applied bias voltage ( V DC ) and measured current ( I DC ) are denoted above the eye diagrams at each temperature. The extinction ratio (ER) and insertion loss (IL) are denoted below the eye diagrams at each data rate and temperature. ( f ) The TDR measurement of the electro-optic modulator energy consumption and switching energy for a 0.5 V PP drive is shown for the indicated DC bias voltages. ( g ) The breakdown of the thermo-optic, electro-optic and total modulator energy consumption is plotted as a function of temperature, showing the 1 fJ bit operation over 7.5 °C temperature range. Full size image Integrating the modulator into a communication link Finally, it is useful to consider the modulator performance in the context of a fully integrated communication link including the driver circuitry. A key part of this consideration is the inclusion of the circuitry that will be necessary to correct for thermal effects. Within a microprocessor, baseline temperature variations are typically within ±5 °C [32] , hence the reason for the comparison of the modulators across a 10 °C range. Over this range, our modulator consumes a total of 2.77 fJ per bit. However, with either a slight reduction in temperature variations on a microprocessor, or with a reduction in the leakage current of our device, 1 fJ per bit operation can be maintained. Moreover, even without these improvements with the use of barrel-shifting techniques [28] , compensation across much broader temperature ranges can be achieved while staying in the 1-fJ per bit electro-optic regime. Indeed, it is only necessary to be able to shift each ring by the channel spacing. Implementation of this technique, however, adds overhead to the power consumption, and this overhead is given by: ~A × log 2 N , where N is the total number of resonators and A is the 2-by-1 electrical multiplexer energy consumed at the given CMOS node (Michael Georgas, Chen Sun, personal communication, 10 April 2014). For the 45, 32, 22 and 11 nm CMOS nodes, the estimated energy consumption of this technique for 86 resonant modulators (71 active and 15 redundant) with a channel spacing of 75 GHz will be 17.88 fJ per bit, 9.9 fJ per bit, 4.3 fJ per bit and 1.3 fJ per bit, respectively [33] , which is expected to scale to <1 fJ per bit below the 10 nm node [34] . In addition to the barrel-shifting circuitry, one must also account for the modulator control circuitry. This circuitry includes the modulator driver, the feedback loop and a monitor receiver, as shown in Fig. 6a . Here, the receiver, attached to a weak drop port, constantly monitors the modulator output and the feedback loop processes that output and locks the modulator to the laser line by adjusting the DC bias of the modulator driver as described in the preceeding paragraph. The energy consumption of such a modulator driver and a monitor receiver were experimentally measured on a 45-nm CMOS node to be 20 and 69 fJ per bit, respectively, (assuming a receiver responsivity of ~1 AW −1 ) [35] . The energy consumption of the feedback loop was also measured on a 180-nm CMOS node to be 0.43 mW (for example, 17.2 fJ per bit at 25 Gb s −1 operation) [36] . It is important, however, to note two things. First, in previous low-power modulators, which rely on thermal tuning, the lowest thermal tuning of ~175 fJ per bit at 25 Gb s −1 still clearly dominates over the driving circuitry in the energy consumption budget. In contrast, for the modulator presented in this work, the circuit energy consumption now dominates the overall energy consumption, an important achievement. Second, current CMOS power consumption is technological, not fundamental, at this level as is shown in Fig. 6b . Among other things, given the CMOS energy consumption scaling [34] , we can see that the driver will consume <1 fJ per bit at or below the 10-nm CMOS node and the total circuit including feedback and the barrel shifter will consume <1 fJ per bit below the 4-nm CMOS node. We therefore expect that with improvements in CMOS technology, the total modulator plus driver circuit energy consumption can be kept in the 1 fJ per bit range for this device. 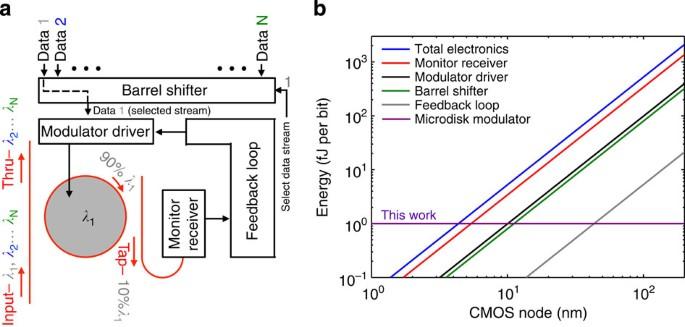Figure 6: Integrated modulator components and energy scaling. (a) A diagram of the required integrated electrical circuitry to drive, and control the modulator and barrel shifter to correct for channel hopping between modulators. (b) The energy consumption scaling of the modulator subsystem is plotted as a function of CMOS node scaling, showing sub-fJ per bit driver and total electronics energy at advanced CMOS nodes. Figure 6: Integrated modulator components and energy scaling. ( a ) A diagram of the required integrated electrical circuitry to drive, and control the modulator and barrel shifter to correct for channel hopping between modulators. ( b ) The energy consumption scaling of the modulator subsystem is plotted as a function of CMOS node scaling, showing sub-fJ per bit driver and total electronics energy at advanced CMOS nodes. Full size image Demonstrating bandwidth-limited transmission In order to demonstrate the highest speed digital operation of the modulator, a voltage amplifier and a bias tee with a 3-dB bandwidth of 40 GHz were attached to the high-speed electro-optic setup (see the Methods section for details) and a 2.2-V PP drive signal with −0.5 V DC bias was delivered to the modulator. High-speed optical eye diagrams, shown in Fig. 7 , were measured with a digital sampling oscilloscope at data rates of up to 44 Gb s −1 . The dynamic ER and IL are shown below each eye diagram in Fig. 7 . With low IL (0.9 dB) and high ER (8.0 dB), the eye diagrams are still open at 44 Gb s −1 . There are a couple of points to consider that enabled this result. The NRZ 44 Gb s −1 data stream only requires ~22 GHz (half of the bit rate) of bandwidth since the spectrum of the NRZ signal is proportional to sinc 2 ( f ), where f is the frequency at the bit rate and the major spectral components are below half of the bit rate [37] . Also, while the electro-optic 3 dB bandwidth was measured to be 21 GHz with a small-signal drive (50 mV PP ), when the modulator is driven at a reverse-biased voltage of −2.2 V, the modulator bandwidth increases to 22.4 GHz due to the reduction in average device capacitance, measured by TDR (see below and Fig. 5f ), from ~16 to ~14 fF. The reduction in device capacitance stems from the increased depletion width at higher reverse bias, also observed in [19] . Finally, the modulator starts to operate in the optically limiting regime at this higher drive voltage, also observed in [19] . In this regime, the optical resonance limits the data levels to the optical ‘0’ and ‘1’, which enables relatively faster transitions. This demonstration shows that the modulator can provide on-demand bandwidth with a measured energy consumption of 17.4 fJ per bit (see the Methods section for details). 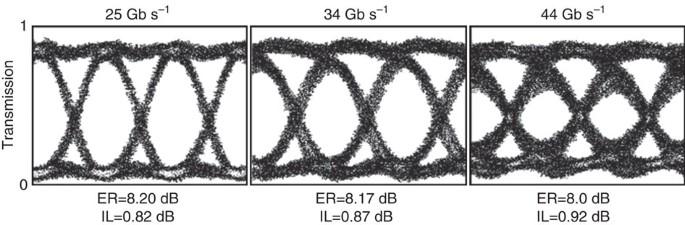Figure 7: Bandwidth-limited data transmission. The experimentally measured high-speed optical eye diagrams of the silicon microdisk modulator when driven by a terminated probe and a 2.2 VPPNRZ-OOK PRBS with a pattern length of 231-1 at data rates of 25-, 34- and 44 Gb s−1. The extinction ratio (ER) and insertion loss (IL) are denoted below the eye diagrams at each data rate. Figure 7: Bandwidth-limited data transmission. The experimentally measured high-speed optical eye diagrams of the silicon microdisk modulator when driven by a terminated probe and a 2.2 V PP NRZ-OOK PRBS with a pattern length of 2 31 -1 at data rates of 25-, 34- and 44 Gb s −1 . The extinction ratio (ER) and insertion loss (IL) are denoted below the eye diagrams at each data rate. Full size image In conclusion, we have demonstrated an athermal silicon photonic modulator with the largest electro-optic response, lowest power and lowest single-ended voltage demonstrated to date. The record 250 pm V −1 (30 GHz V −1 ) electro-optic response enables error-free 0.9 fJ per bit operation at a data rate of 25 Gb s −1 with an AC-coupled drive of 0.5 V PP in a 4.8-μm diameter microdisk modulator. Further, the large response leads to a small parasitic (0.24 fJ per bit) tuning energy consumption but when combined with a reduction in the modulation energy consumption to 0.79 fJ per bit at the compensated temperature, leads to a total energy consumption of 1.03 fJ per bit over a 7.5 °C temperature range. Over a 10 °C temperature range, the increased leakage current increases the tuning energy consumption to 2 fJ per bit, while sustaining error-free 0.77 fJ per bit operation at a data rate of 25 Gb s −1 for a total energy consumption of 2.77 fJ per bit. Driven harder, the modulator demonstrates open-eye diagrams out to 44 Gb s −1 . The electro-optic response of the circularly contacted vertical junction device is up to 10 times larger than that achieved with lateral junction-based modulators, thus enabling both efficient modulation and the electro-optic control of the resonant frequency. The combined result improves upon the overall energy consumption of modulators by nearly two orders of magnitude. No other resonant modulator today is capable of achieving a similar result. Yet, these results represent only the beginning of electro-optic control of the resonant frequency. Future modulators and filters with maximized capacitance per unit volume (for example, in multiple vertical junctions such as an n–p–n junction or perhaps high spatial frequency interleaved junctions [38] ) in a smaller footprint will clear the way for direct control of even greater temperature variations with even less leakage current. While the modulator represents only one component of a silicon photonic link, as photonics becomes more closely integrated with CMOS, and as the bandwidth requirements on- and off-chip continue to rise, the power consumption of each component will be pressed to achieve new levels of efficiency in order to fit within the overall power envelope of the communication link. With their efficient 1 fJ per bit operation at the increasingly important 25 Gb s −1 data rate, and with the effective elimination of heater power consumption, these results represent an important first step towards achieving femtojoule per bit class communication links that will prove critical for future on-chip applications. Device fabrication The microdisk modulator was fabricated in a 300-mm CMOS foundry with a 65-nm technology node, using silicon-on-insulator wafers with a 0.225-μm top silicon layer and 2-μm buried oxide layer for optical isolation. A full silicon etch was applied to form the silicon resonant microdisk and bus waveguides. An oxidization step followed to passivate the sidewalls, which also decreased the waveguide thickness to 0.22 μm. The vertical junction, centered slightly above 110 nm thickness, was formed from arsenic (As) and boron difluoride (BF 2 ) implants with designed doses of 4 × 10 13 and 2.77 × 10 13 cm −2 , and energies of 380 and 120 keV, respectively. Through fitting the experimental spectral response of the modulator as a function of voltage, the As and BF 2 implants were determined to be formed with equivalent energies of 415 and 90 keV, respectively. The overlapping n+ and p+-doped regions in the center of the microdisk were formed from phosphorus and BF 2 implants with doses of 5 × 10 15 and 3.5 × 10 15 cm −2 , and energies of 180 and 120 keV, respectively. The target p-type and n-type doping concentrations were both 2.5 × 10 18 cm −3 and p+ and n+-type doping concentrations were >2 × 10 20 cm −3 . An oxide (SiO 2 ) layer with a total thickness of 3.6 μm was deposited to cover the modulator. Low-resistance contacts to p+ and n+-doped regions were made by standard silicidation, copper-silicon circular and point contacts. Finally, the contacts were connected to on-chip ground-signal-ground (GSG)-probing pads by two metal layers. Numerical simulation The carrier distribution as a function of voltage, simulated by Sentaurus, was converted into an index distribution using the plasma dispersion (electro-refraction) equations in refs 14 , 22 . The index distribution was fed into the FDM [26] to determine the complex propagation constant as a function of voltage. The complex propagation constant was then input to the transfer matrix of the resonant modulator [39] in order to theoretically predict the spectral response as a function of voltage. Time domain reflectometer measurement The absorbed power of the modulator was determined by subtracting two TDR measurements. First, the reflected voltage ( V P − ) from the transmission line, non-terminated GSG probe and pads ( Z P ) was initially determined using the experimental setup, shown in Fig. 3a . The reflected voltage was then normalized to the emanating step voltage ( V in ) to extract the frequency domain reflection coefficient, , where, Z 0 , 50 Ω, is the characteristic impedance of the transmission line. The absorbed switching power in this path was determined by the following equation, . Second, the reflected voltage ( V PM − ) from this path and the modulator ( Z M ), connected to the identical wiring, was determined using the experimental setup, shown in Fig. 3b . The normalized frequency domain reflection coefficient and absorbed switching power was determined by the following equations, and , respectively. With close electrical and photonics integration these devices will not require long transmission lines, probing or large GSG pads. Therefore, the absorbed power of stand-alone modulator is , which can be calculated by subtracting the previously measured power consumptions, . The switching power of the modulator ( P s m ) was integrated over time to obtain switching energy, . The exact switching energy using the above equation was determined to be 3.65 fJ (0.91 fJ per bit). Alternatively, using the parallel equivalent impedance model, , we can approximate the modulator reflection coefficient with the following equation: which was also performed in ref. 14 . This approximation is accurate for Z P >> Z 0 2 , and overestimates the high frequency power consumption as Z P approaches to Z 0 2 . The approximated switching energy using the above equations was determined to be 3.84 fJ (0.96 fJ per bit), which is in good agreement with the exact switching energy. High-speed electro-optic setup The electrical data, encoded using a pattern generator, was a NRZ on-off-keyed signal, encoded with a 2 31 –1 PRBS. The output of the pattern generator was 0.5 V PP with a +0.25 V DC bias, and a DC block was attached to achieve an AC-coupled 0.5 V PP drive. A 50-Ω-terminated GSG probe was used to eliminate transmission line reflections and ensure that the voltage dropped across the modulator was 0.5 V PP . This termination is not required when electronics are integrated on-chip since wire lengths will be on the order of 10–100μm, where transmission line effects are negligible for wires up to a millimetre in length ( λ RF /10, where λ RF =10 mm) at 25 Gb s −1 operation. The laser line, coupled into the microdisk, was set to λ ~1,587.4 nm and the through port output was then passed through an erbium-doped fibre amplifier (EDFA) to overcome fibre-to-chip coupling losses. A tunable bandpass filter with a 1-nm 3-dB bandwidth was used to filter out the amplified spontaneous emission of the EDFA. In addition, a variable optical attenuator was inserted before the high-speed p – i – n photodiode and transimpedance amplifier receiver. The received data were then fed differentially to a BER tester for evaluation. No pre-emphasis or equalization of the signal was used throughout the measurements. The total fibre-to-fibre IL was ~14.5 dB, and the intensity before the EDFA was ~−9 dBm. Temperature-controlled setup In order to alter and record the chip temperature, a thermoelectric-cooler (TEC) was attached to the silicon substrate and a thermistor, placed adjacent to the silicon chip, was used to feedback the temperature readout. Then, a commercial TEC proportional-integral-derivative controller was used to stabilize the chip temperature from 20 to 30 ° C with ±0.05 ° C accuracy. The continuous-wave laser was set to λ ~1,587.6 nm and fibre-to-chip coupling optimized for each temperature set point due to the thermal expansion of the TEC. How to cite this article : Timurdogan, E. et al. An ultralow power athermal silicon modulator. Nat. Commun. 5:4008 doi: 10.1038/ncomms5008 (2014).